Electrical magnetochiral anisotropy in a bulk chiral molecular conductor So far, no effect of chirality on the electrical properties of bulk chiral conductors has been observed. Introduction of chiral information in tetrathiafulvalene precursors represents a powerful strategy towards the preparation of crystalline materials in which the combination of chirality and conducting properties might allow the observation of the electrical magnetochiral anisotropy effect. Here we report the synthesis by electrocrystallization of both enantiomers of a bulk chiral organic conductor based on an enantiopure tetrathiafulvalene derivative. The enantiomeric salts crystallize in enantiomorphic hexagonal space groups. Single crystal resistivity measurements show metallic behaviour for the enantiopure salts down to 40 K, in agreement with band structure calculations. We describe here the first experimental evidence of electrical magnetochiral anisotropy in these crystals, confirming the chiral character of charge transport in our molecular materials. Chirality manifests itself in many areas of physics, chemistry and biology, where objects or materials can exist in two non super-imposable forms, one being the mirror image of the other [1] . It is easily observed in the optical properties of dielectric materials, as optical activity or circular dichroism. However for conductors, such a characterization is not available and other methods are needed. On the basis of symmetry arguments, Rikken et al. [2] have argued that the two-terminal electrical resistance of a chiral conductor subject to a magnetic field B is of the form where I is the electrical current. Parity reversal symmetry requires for the magnetochiral anisotropy parameter γ D =−γ L where D and L indicate the right- and left-handed version of the conductor, respectively [2] . We neglect higher-order symmetry-allowed terms that are odd order products of each B and I, similar to I·B 3 . The parameter β describes the normal magnetoresistance that is allowed in all conductors. Here we neglect higher even orders in B that are also allowed. We call the effect corresponding to the linear B dependence in equation 1 electrical magnetochiral anisotropy (eMChA), in direct analogy to the optical case [3] , which corresponds to a polarization-independent enantioselective contribution to the optical properties of chiral media that depends on the relative orientation of the direction of light and magnetic field. The existence of these effects is the direct consequence of the simultaneous breaking of time-reversal symmetry by a magnetic field and of parity by chirality and is therefore fundamental and universal. We can quantify the eMChA by Δ R ( I , B )≡ R ( I , B )− R (– I , B ) from which follows This effect was observed for the first time in a model system consisting of bismuth helices, with γ =10 −3 T −1 A −1 (ref. 2 ), followed by its observation in individual single-walled carbon nanotubes at low temperatures with γ =10 2 T −1 A −1 (ref. 4 ), the latter value being in reasonable agreement with model calculations [5] . Both the experimental and theoretical results on carbon nanotubes were later on independently confirmed [6] , [7] , [8] , [9] . If we rephrase the eMChA in terms of the magnetization M of the medium, it also covers the case of the transmission of spin-polarized electrons through chiral gases [10] or through chiral DNA layers [11] as manifestations of eMChA, thus creating a link between chirality and spintronics [12] . It would also predict similar observations for ferromagnetic chiral conductors [13] in the absence of an external magnetic field. The double phase-sensitive detection used for the earlier observations is limited to Δ R / R ~10 −6 (ref. 2 ). Therefore, we have developed a new heterodyne method to detect very small magnetochiral anisotropies (see Supplementary Note 1 ). In the most favourable cases, a detection limit of Δ R/R ≈10 −9 was obtained with this heterodyne method, which allows observation of eMChA at much lower currents than before. So far, eMChA has not been observed in a bulk chiral conductor. The symmetry arguments evoked above evidently apply, and the effect should exist in such systems, which should be quite abundant (of the 230 crystal space groups, 65 are chiral) but which can rarely be obtained in a well-defined enantiopure form. No detailed theory of charge transport in bulk chiral conductors has been formulated so far. In such materials, the trajectories of the charge carriers can be strongly randomized by scattering, effectively reducing their coupling to the chiral crystal structure, and the orbital contributions to the eMChA effect are expected to be weaker than in conductors that are geometrically chiral. Spin contributions should be less affected by scattering, unless spin-orbit coupling or magnetic scatterers are present. Chirality may also affect bulk band structure parameters, as Fermi velocities. As eMChA is the only known manifestation of chirality in chiral conductors, we have set out to look for this effect in bulk chiral conductors. Tetrathiafulvalene (TTF) and its derivatives represent the most important family of electroactive precursors extensively used for the preparation of bulk crystalline molecular conductors and superconductors [14] . Although the first chiral TTF, namely the ( S,S,S,S ) enantiomer of tetramethyl-bis(ethylenedithio)-TTF (TM-BEDT-TTF), has been synthesized in the middle 80s (ref. 15 ), only much more recently there has been an increasing interest in the introduction of chiral information in TTF derivatives [16] , mainly motivated by the possible detection of the eMChA effect. Nevertheless, as mentioned earlier, no such evidence has been provided so far in bulk conductors, including the TTF-based materials, although the influence of chirality on the conducting properties of TTF conductors has been indirectly expressed through the modulation of the structural disorder in a few series of conducting radical cation salts based on chiral TTF-oxazoline [17] , [18] or TM-BEDT-TTF donors [19] , in which the enantiopure materials were more conducting than the racemic ones because of the structural disorder present in the latter. Compared with the relatively large number of chiral TTF precursors [16] , [20] , only a few examples of derived conducting materials have been described, such as those based on TM-BEDT-TTF [13] , [19] , [21] dimethyl-bis(ethylenedithio)-TTF (DM-BEDT-TTF) [22] , [23] , or TTF-oxazoline [17] , [18] . Moreover, complete series of conducting salts containing both enantiomers and the racemic forms, in order to compare their conducting properties, are even more scarce [17] , [18] , [19] , and in all of them the enantiomeric pairs crystallize within the same space group, although there is in principle the possibility that enantiomers crystallize in one of the 11 enantiomorphic space groups, which remains, however, a relatively rare event. We have recently used the so far unexplored dimethyl-ethylenedithio-TTF (DM-EDT-TTF) donor in electrocrystallization experiments, which provided a first family of radical cation salts formulated as (DM-EDT-TTF) 2 PF 6 , with semiconducting properties for the enantiopure compounds, while the racemic form shows metallic behaviour [24] . In the present work, we select the chiral salts (DM-EDT-TTF) 2 ClO 4 as candidates for the eMChA effect in bulk conductors. We describe herein their synthesis, solid-state structures and physical properties supported by band structure calculations. Synthesis and crystal structures of the chiral salts Single crystals of both handedness were prepared by electrocrystallization of enantiopure ( S,S )- or ( R,R )-DM-EDT-TTF ( 1 and 2 , Fig. 1 ) in the presence of (NBu 4 )ClO 4 as supporting electrolyte. 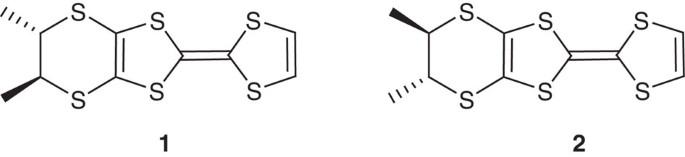Figure 1: Enantiopure DM-EDT-TTF donors. (S,S)-DM-EDT-TTF (1) and (R,R)-DM-EDT-TTF (2). Figure 1: Enantiopure DM-EDT-TTF donors. ( S,S )-DM-EDT-TTF ( 1 ) and ( R,R )-DM-EDT-TTF ( 2 ). Full size image The salts are formulated as (DM-EDT-TTF) 2 ClO 4 and they crystallize, very interestingly, in the enantiomorphic hexagonal space groups P6 2 22 and P6 4 22 for the ( S,S ) and the ( R,R ) enantiomers, respectively, with one independent half of donors and a quarter of anions in the asymmetric unit ( Supplementary Table 1 ). This represents the first enantiomeric pairs of radical cation salts crystallizing in enantiomorphic space groups. The donors show planar geometry, with the methyl substituents disposed in equatorial positions ( Fig. 2 and Supplementary Fig. 1 ). 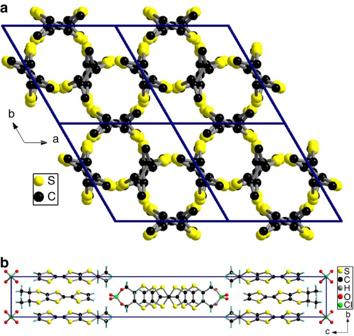Figure 2: Crystal structure of [(S,S)-DM-EDT-TTF]2ClO4. (a) Packing diagram of [(S,S)-DM-EDT-TTF]2ClO4in theabplane with an emphasis on the hexagonal symmetry (H atoms and ClO4anions have been omitted for clarity). (b) Lateral view in thebcplane. Figure 2: Crystal structure of [( S,S )-DM-EDT-TTF] 2 ClO 4 . ( a ) Packing diagram of [( S,S )-DM-EDT-TTF] 2 ClO 4 in the ab plane with an emphasis on the hexagonal symmetry (H atoms and ClO 4 anions have been omitted for clarity). ( b ) Lateral view in the bc plane. Full size image Bond length values, in particular the central C=C and internal C–S bonds ( Supplementary Table 2 ), are in agreement with the mixed valence state of +0.5 per donor molecule, as indicated by the 2:1 stoichiometry of the salt. The donors pack along the b direction with the formation of uniform chains that interact laterally through short S···S contacts ( Supplementary Fig. 2 ). The hexagonal axis corresponds to the c direction that encompasses the successive donor and anion layers, and thus the donors are rotated from one layer to the next one by 120° clockwise or anticlockwise, depending on their handedness ( Fig. 2 ). The chirality of the donor is thus transposed at the crystal level. The oxygen atoms of the anion are involved each in one H vinyl ···O and one H Me ···O hydrogen bonds measuring 2.69 and 2.68 Å, respectively ( Supplementary Fig. 3 ). Electrocrystallization of the racemic mixture of DM-EDT-TTF affords the racemic salt (DM-EDT-TTF)ClO 4 , which crystallizes in the monoclinic system, centrosymmetric space group P2 1 /c . The donors thus bear a charge +1 and form strong head-to-tail dimeric units with short intramolecular S···S contacts ( Supplementary Figs 4 and 5 ). This time the methyl groups occupy axial positions. Band structure calculations The mixed valence state of the enantiopure salts together with their peculiar crystalline symmetry and packing represent a favourable situation for good transport properties in these chiral materials, which prompted us to perform band structure calculations. In the following only the results for the ( R,R ) enantiomer are presented since those for the ( S,S ) one (see Supplementary Note 2 and Supplementary Figs 6 and 7 ) are similar. The donor layers of the salt contain one symmetry non-equivalent donor and two different donor···donor interactions, one along the stack (I) and one along the interstack direction (II; Fig. 3 ). 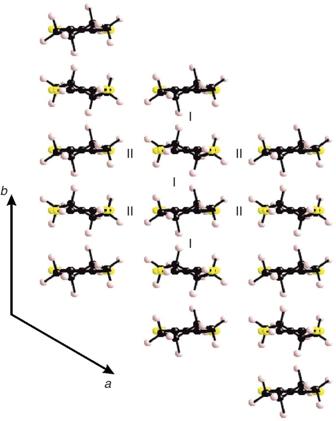Figure 3: Packing of donors. Donor layer of the[(R,R)-DM-EDT-TTF]2ClO4salt. Figure 3: Packing of donors. Donor layer of the [( R,R )-DM-EDT-TTF] 2 ClO 4 salt. Full size image Both |β HOMO–HOMO | interaction energies, which are a measure of the strength of the HOMO···HOMO interactions determining the band structure near the Fermi level, are strong—that is, 0.4031, eV (I) and 0.2090, eV (II) ( Supplementary Tables 3 and 4 ), although those along the stacks are twice larger. Note that the S···S contacts are considerably shorter for the interstack interaction. These contacts are however of the weaker lateral π-type, whereas those associated with the intrastack interaction are of the stronger σ-type. Hence, as far as the HOMO···HOMO interactions are concerned, the system should be considered as a series of quite significantly coupled uniform chains, and thus a large dispersion of the HOMO bands is anticipated. Because of the stoichiometry the two HOMO bands must contain one hole and consequently the upper band is half-filled. These two observations lead to the prediction that the system should be metallic. The calculated band structure is shown in Fig. 4a . As expected, the HOMO bands exhibit dispersion along all directions and a quite large total dispersion is found. The two bands are degenerate at the Y point because of the existence of screw axis parallel to the b direction—that is, the stacks direction. Note however that the dispersion of the partially filled band is not that different along a * and b *, something which could seem to be at odds with the fact that the strength of the HOMO···HOMO interaction is twice larger along the stack’s direction. The reason is that because of the 120° angle between the a and b axes, while moving from Γ to X ( a */2, 0) or Y (0, b */2) both the intrachain and interchain interactions are changing and they partially compensate or reinforce along the lines shown in Fig. 4a . The important point to notice is that the Fermi level cuts the Γ→Y line near the Γ point but does not cut the Γ→X line. This means that the system must exhibit an open, although quite warped, Fermi surface perpendicular to the stack direction. Consequently, the layers should behave as a pseudo-one-dimensional metal along the stack direction. The chirality of the crystal should express itself in this warping; however, so far this aspect is beyond our means. 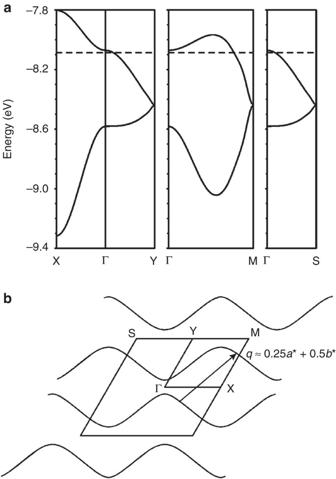Figure 4: Electronic band structure and Fermi surface. (a) Calculated band structure for the donor layers of the[(R,R)-DM-EDT-TTF]2ClO4salt. The dashed line refers to the Fermi level and Γ=(0, 0), X=(a*/2, 0), Y=(0,b*/2), M=(a*/2,b*/2) and S=(−a*/2,b*/2). (b) Calculated Fermi surface. Theqvector shown in is the nesting vector of the Fermi surface. Figure 4: Electronic band structure and Fermi surface. ( a ) Calculated band structure for the donor layers of the [( R,R )-DM-EDT-TTF] 2 ClO 4 salt. The dashed line refers to the Fermi level and Γ=(0, 0), X=( a */2, 0), Y=(0, b */2), M=( a */2, b */2) and S=(− a */2, b */2). ( b ) Calculated Fermi surface. The q vector shown in is the nesting vector of the Fermi surface. Full size image The calculated Fermi surface is shown in Fig. 4b . It is built from a series of strongly warped open lines perpendicular to the stacks direction ( b ). This Fermi surface exhibits an almost perfect nesting with q≈0.25 a *+0.5 b *. Consequently, the low-temperature abrupt change in the resistivity ( vide infra ) is most probably associated with either a charge or spin density wave modulation with this wave vector, that should completely destroy the Fermi surface and lead to an insulator behaviour. The b * component of the modulation stems from the fact that the band is half-filled and the a * component means that, besides Coulomb interactions between the modulations, the direct interstack interaction favours a new repeat unit with four donor stacks. Single crystal conductivity measurements The band structure calculations are fully supported by the conducting properties of both materials. Accordingly, single crystal resistivity measurements show conducting behaviour for [( S,S )-DM-EDT-TTF] 2 ClO 4 and [( R,R )-DM-EDT-TTF] 2 ClO 4 with room temperature conductivity values between 10 and 20 S cm –1 . Both compounds show an abrupt metal to insulator (MI) transition at around 40 K ( Supplementary Fig. 8 ). The temperature of the transition is gradually shifted down under an applied hydrostatic pressure, T MI ≈15 K for P =11 kbar ( Supplementary Fig. 9 for ( S , S ) and Fig. 10 for ( R , R )), but not totally suppressed. As discussed above, the observed MI transition can be related to a spin or charge density modulation as suggested by the possible nesting of the Fermi surface. As expected from the X-ray analysis—that is, 1:1 stoichiometry and strong dimerization of the donors—the resistivity of the [( rac )-DM-EDT-TTF]ClO 4 salt at room temperature is high (10 6 Ω m) and its temperature dependence is activated ρ=ρ 0 exp(E a /T), with a very high activation energy: E a =7,000 K (0.6 eV; Supplementary Fig. 11 ). eMChA effect With the two enantiomeric salts of DM-EDT-TTF available, we have unique candidates for the investigation of the eMChA effect in bulk conductors, since they are metallic at room temperature and ambient pressure, and, moreover, the individual chirality of the donors is expressed to the crystal level through the formation of enantiomorphic crystals. Typical dimensions of the crystals were 1 × 0.3 × 0.1 mm 3 ( Supplementary Figs 12 and 13 ), with the long axis along the crystal b axis, which is also the current- and the magnetic field direction. The resistivity of the material as determined by four terminal measurements was around 10 −3 Ω m, in agreement with values mentioned above. Typical results for the current and magnetic field dependence of the magnetochiral anisotropy at room temperature, obtained by the heterodyne method in a four-terminal configuration and expressed as the eMChA voltage, are shown in Fig. 5a,c for a (R,R) enantiomer crystal. The top panel ( Fig. 5a ) confirms the linear dependence of this eMChA voltage on the magnetic field; the bottom panel ( Fig. 5c ) shows the quadratic dependence of this voltage on the current, together confirming the linear dependence of the relative resistance anisotropy ΔR / R on current and field. Crystals of the ( S , S ) enantiomer show dependencies on current and field of the opposite sign but with magnitudes that were of the same order ( Fig. 5b,d ). It should be noted that at the highest currents that could be used, a superlinear (but still odd) magnetic field dependence seems to develop for both samples but is more pronounced for the ( S,S ) sample. We currently have no explanation for this observation, other than that it is symmetry-allowed. The results obtained for different crystals are summarized in Table 1 , where we have only used the lowest field results in the top panels to extract the γ values (solid lines), instead of all results (dashed lines). The fact that we find γ values that are very similar for all crystals lends credibility to this procedure. 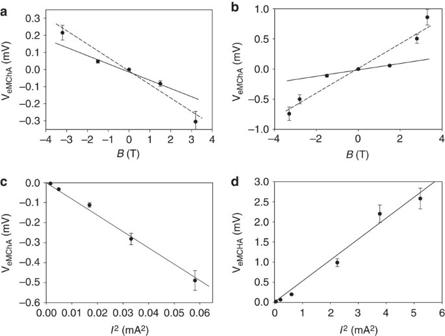Figure 5: eMChA results. The results shown were obtained on the sample [(R,R)-DM-EDT-TTF]2ClO4–B (a,c) and the sample [(S,S)-DM-EDT-TTF]2ClO4–A (b,d).γ=VeMChA/2GRBI2, where G is a preamplifier gain, equal to 185. (a,b) Show the odd dependence of the effect on the magnetic field. (c,d) Panels show the quadratic dependence of the heterodyne voltage on the current, which translates to a linear current dependence of the eMChA. Straight lines are linear fits (see text), error bars correspond to variations between consecutive measurements. Figure 5: eMChA results. The results shown were obtained on the sample [( R , R )-DM-EDT-TTF] 2 ClO 4 –B ( a , c ) and the sample [( S , S )-DM-EDT-TTF] 2 ClO 4 –A ( b , d ). γ =V eMChA /2GRBI 2 , where G is a preamplifier gain, equal to 185. ( a , b ) Show the odd dependence of the effect on the magnetic field. ( c , d ) Panels show the quadratic dependence of the heterodyne voltage on the current, which translates to a linear current dependence of the eMChA. Straight lines are linear fits (see text), error bars correspond to variations between consecutive measurements. Full size image Table 1 Summary of the different samples measured. Full size table Attempts to do eMChA measurements at lower temperatures so far failed because of contact problems but will be further pursued. A quantitative comparison of the eMChA results for the bismuth helices [2] , the SWCNT [4] and [DM-EDT-TTF] 2 ClO 4 is not straightforward as they are of very different nature. One can quantify the experimental results for the eMChA in terms of the current as defined above, but also in terms of the average current density J as in Table 2 summarizes the different results expressed in these two manners, which give very different relative strengths between the three different systems. Table 2 Typical parameters for equations 1 and 4, for different systems. Full size table To our knowledge, no microscopic theory for eMChA in bulk chiral conductors has been developed so far. The two microscopic mechanisms identified as causes for eMChA in the model system of bismuth helices were the current induced magnetic field in combination with the magnetoresistance (the β term in equation 1) and scattering by screw dislocations [2] . The smallness of β and the good crystalline quality seem to rule out these mechanisms for [DM-EDT-TTF] 2 ClO 4 . The helix model of carbon nanotubes identified enantioselective current- and field dependent differences in Fermi velocity v F and density of states at the Fermi level n F as dominant mechanisms for eMChA in SWCNT [4] , which was confirmed by de Martino (ref. 9 ) in a more realistic approximation. The eMChA parameter γ expressing the relative anisotropy, such mechanisms would allow for a large γ in metals where v F and n F are low, as is the case of most organic metals [25] like [DM-EDT-TTF] 2 ClO 4 . It seems therefore a reasonable hypothesis that the same mechanisms are responsible for eMChA in [DM-EDT-TTF] 2 ClO 4 . In conclusion, the eMChA effect has been observed for the first time in the case of bulk metallic chiral conductors. Opposite in sign, but equal in magnitude, field and current dependencies of the anisotropy factors are shown for the enantiomeric salts ( S , S ) and ( R , R ) [DM-EDT-TTF] 2 ClO 4 prepared by electrocrystallization. Their single crystal X-ray analyses evidence that they crystallize in the enantiomorphic hexagonal space groups P6 2 22 and P6 4 22 , respectively. Although a theoretical model explaining the mechanism of eMChA in bulk conductors has still to be formulated, our results open the way towards the study of this phenomenon in other TTF based chiral conductors and superconductors. The case of chiral superconductors is particularly intriguing as eMChA lifts the degeneracy between electrons moving with wavevectors k and – k , which are the building blocks of Cooper pairs and thereby of superconductivity. As eMChA can be regarded as a spin filtering effect, an obvious link with spintronics exists, a topic that so far has not involved organic conductors. Sample preparation The enantiopure donors ( S,S )-DM-EDT-TTF and ( R,R )-DM-EDT-TTF have been prepared as recently described [24] . Electrocrystallization experiments were carried out under argon; dry tetrahydrofuran was obtained from distillation machines; 1,1,2-dichloroethane was purchased from Aldrich and used as freshly distilled. Dark-black single crystals of [( S,S )-DM-EDT-TTF] 2 ClO 4 and [( R,R )-DM-EDT-TTF] 2 ClO 4 were obtained by electrocrystallization as follows: 19 mg of [NBu 4 ]ClO 4 were dissolved in 7 ml of a mixture of 1,1,2-trichloroethane: tetrahydrofuran 1:1 and the solution was poured in the cathodic compartment of the electrocrystallization cell. The anodic chamber was filled with 5 mg of donor dissolved in 7 ml of a mixture of 1,1,2-trichloroethane:tetrahydrofuran 1:1. Single crystals of the salt were grown at 2–3 °C over a period of 4 weeks on a platinum wire electrode, by applying a constant current of 1 μA. Black crystalline plates were grown on the electrode. Dark-black single crystals of [( rac )-DM-EDT-TTF]ClO 4 were obtained by electrocrystallization as follows: 19 mg of [NBu 4 ]ClO 4 were dissolved in 7 ml of a mixture of 1,1,2-trichloroethane:tetrahydrofuran 1:1 and the solution was poured in the cathodic compartment of the electrocrystallization cell. The anodic chamber was filled with 5 mg of (rac)- DM-EDT-TTF (2.5 mg of ( S,S ) and 2.5 mg of ( R,R ) enantiomers) dissolved in 7 ml of a mixture of 1,1,2-trichloroethane:tetrahydrofuran 1:1. Single crystals of the salt were grown at 2–3 °C over a period of 2 weeks on a platinum wire electrode, by applying a constant current of 1 μA. Black prismatic crystals were grown on the electrode. X-ray crystallography X-ray diffraction measurements were performed on a Nonius Kappa CCD diffractometer, using graphite-monochromated Mo K α radiation ( λ =0.71073 Å). The structures were solved (SHELXS-97) by direct methods and refined (SHELXL-97) by full-matrix least-square procedures on F 2 . The non-H atoms were refined with anisotropic displacement parameters. A summary of the crystallographic data and the structure refinement is given in Supplementary Table 1 . Band structure calculations The tight-binding band structure calculations [26] were of the extended Hückel type. A modified Wolfsberg–Helmholtz formula was used to calculate the non-diagonal H μν values [27] . All valence electrons were taken into account in the calculations and the basis set consisted of Slater-type orbitals of double-ζ quality for C 2s and 2p, S 3s and 3p and of single-ζ quality for H. The ionization potentials, contraction coefficients and exponents were taken from previous work [28] . Single crystal conductivity measurements For both conducting enantiomers [( S,S )-DM-EDT-TTF] 2 ClO 4 and [( R,R )-DM-EDT-TTF] 2 ClO 4 , a four-point method was used with a low frequency (<100 Hz) lock-in technique using a measuring current I ac =1 μA. Resistivity measurements were performed at ambient pressure and also under high hydrostatic pressure in a CuBe clamped cell up to 12 kbar with silicon oil (Daphne 7373) as the pressure transmitting medium. The pressure at room temperature was extracted from the resistance of a manganin gauge in the pressure cell and it is this value that is indicated in the figures ( Supplementary Figs 9 and 10 ). However, the loss of pressure during cooling is estimated to be 2 kbar. A copper-constantan thermocouple inside the pressure cell was used as the thermometer. The electrical conductivity of the insulating compound [( rac )-DM-EDT-TTF]ClO 4 was recorded at ambient pressure in a two-point configuration, applying a constant voltage of 25 V and measuring the current as a function of temperature. All samples were cooled down to 8 K in a Helium-free cryocooler equipment. Accession codes: The X-ray crystallographic coordinates for structures reported in this Article have been deposited at the Cambridge Crystallographic Data Centre (CCDC), under deposition numbers CCDC 966648 [( S,S )-DM-EDT-TTF] 2 ClO 4 , CCDC 966649 [( R,R )-DM-EDT-TTF] 2 ClO 4 , CCDC 966650 [( rac )-DM-EDT-TTF]ClO 4 . These data can be obtained free of charge from The Cambridge Crystallographic Data Centre via www.ccdc.cam.ac.uk/data_request/cif . How to cite this article: Pop, F. et al. Electrical magnetochiral anisotropy in a bulk chiral molecular conductor. Nat. Commun. 5:3757 doi: 10.1038/ncomms4757 (2014).